Protein conformational dynamics dictate the binding affinity for a ligand Interactions between a protein and a ligand are essential to all biological processes. Binding and dissociation are the two fundamental steps of ligand–protein interactions, and determine the binding affinity. Intrinsic conformational dynamics of proteins have been suggested to play crucial roles in ligand binding and dissociation. Here, we demonstrate how protein dynamics dictate the binding and dissociation of a ligand through a single-molecule kinetic analysis for a series of maltose-binding protein mutants that have different intrinsic conformational dynamics and dissociation constants for maltose. Our results provide direct evidence that the ligand dissociation is determined by the intrinsic opening rate of the protein. Transient interactions between a protein and a ligand are central to all biological processes including signal transduction, cellular regulation and enzyme catalysis. Binding and dissociation of a ligand are the two fundamental steps of ligand–protein interactions. Understanding the molecular mechanisms for the binding and dissociation of a ligand therefore provides fundamental insight into how the biological functions are accurately regulated and controlled through protein–ligand interactions [1] . Traditionally, molecular interactions have been quantified by measuring the dissociation constant ( K d ) or binding affinity (1/ K d ). Many biochemical processes in living cells, however, occur in non-equilibrium conditions, and there has been a growing recognition that the binding rate ( k 1 ) and dissociation rate ( k −1 ) of molecular interactions provide more decisive clues for understanding the cell physiology resulting from molecular interactions. For instance, the residence time of a ligand has a significant effect on the signal transduction, regulatory processes and drug responses [2] , [3] , [4] , [5] . Non-covalent interactions between a protein and a ligand at an interface have been considered to be major forces driving the binding and dissociation of a ligand. In many protein–ligand interactions, however, the structural rearrangements of a protein and a ligand usually follow the ligand binding [6] , [7] , [8] . Furthermore, recent studies have revealed protein dynamics that transiently sample a structure similar to the ligand-bound form in the absence of a ligand, raising the question of what crucial roles the protein dynamics play in the binding and dissociation of cognate ligands [9] , [10] , [11] . In a popular view, termed the conformational selection model, ligand binding was proposed to be strongly coupled to protein dynamics; a ligand selectively binds to a subset of a conformational ensemble, similar to the ligand-bound form, and shifts the equilibrium [9] . However, our recent single-molecule fluorescence resonance energy transfer (smFRET) study on maltose-binding proteins (MBPs) revealed that the presence of conformational dynamics does not dictate the ligand-binding step [12] , leaving the role of protein dynamics in the ligand dissociation an open question. Here, we demonstrate how protein dynamics dictate the ligand dissociation, and consequently the binding affinity, by a kinetic analysis of the conformational changes in the mutants of a MBP using smFRET measurements. The MBP mutants were constructed through mutations in the hinge region to have different dissociation constants ( K d ) for maltose, while their ligand-binding interfaces remain intact, providing a perfect model to investigate the role of conformational dynamics in the ligand dissociation and binding affinity. Construction of MBP mutants with varying binding affinities Hinge mutations of MBP are known to significantly alter the binding affinity while maintaining the ligand-binding interfaces [13] , [14] . We constructed a series of MBP mutants by replacing the amino-acid residues at positions 96 and 329 in the hinge region of a protein ( Fig. 1a ) with larger or smaller amino acids ( Fig. 1b ). 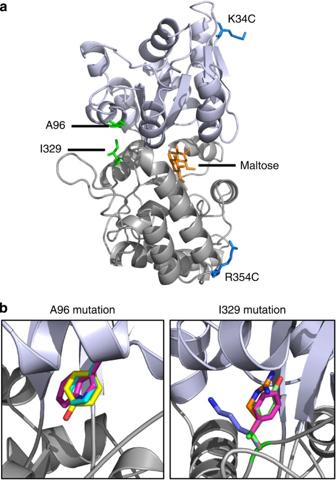Figure 1: Structure and mutation sites of an MBP. (a) MBP mutants with different binding affinities for maltose were constructed by changing the amino-acid residues at two positions, 96 and 329, in the hinge region of the protein (PDB ID code 3MBP), opposite the maltose-binding site of the MBP. Two cysteine residues were introduced into K34/R354 for the labelling of a FRET pair (Cy3 and Cy5). (b) Two sites for mutations in the hinge region of the MBP. Target residues for hinge mutations are marked, and mutated residues (Trp, Tyr, Phe or Tyr, Phe, Arg, Lys) are typically shown in either site of A96 and I329. Isothermal titration calorimetry (ITC) experiments showed that the binding affinities of the mutants for maltose have a strong dependence on the side-chain volume of the amino-acid residues at positions 96 and 329 ( Table 1 ; Supplementary Fig. 1 ), resulting in a two orders of magnitude variation in the dissociation constant. Replacement of the amino-acid residues at position 329 with those with a bulky hydrophobic group (Trp, Tyr and Phe) resulted in a more significant increase in the binding affinity than at position 96. The mutation of isoleucine to tyrosine at position 329 led to the highest binding affinity for maltose. On the other hand, mutations to smaller amino-acid residues such as alanine generally caused a decrease in the binding affinity. Figure 1: Structure and mutation sites of an MBP. ( a ) MBP mutants with different binding affinities for maltose were constructed by changing the amino-acid residues at two positions, 96 and 329, in the hinge region of the protein (PDB ID code 3MBP), opposite the maltose-binding site of the MBP. Two cysteine residues were introduced into K34/R354 for the labelling of a FRET pair (Cy3 and Cy5). ( b ) Two sites for mutations in the hinge region of the MBP. Target residues for hinge mutations are marked, and mutated residues (Trp, Tyr, Phe or Tyr, Phe, Arg, Lys) are typically shown in either site of A96 and I329. Full size image Table 1 Mutated residues and dissociation constants ( K d ) of MBP mutants. Full size table Intrinsic conformational dynamics of MBP mutants We first attempted to determine the intrinsic conformational dynamics of the mutants in the absence of a ligand using smFRET measurements. For this, we labelled MBP mutants with a biotin at its N terminus, and introduced cysteine residues at two positions (Lys34 and Arg354) for conjugating a FRET pair (Cy3 and Cy5) ( Fig. 1a ). The dye-labelling positions were shown to be sensitive enough such that significant changes in the FRET efficiency ( E FRET ) arose during the conformational transitions between the apo- and holo-forms [12] . An amylose-binding assay and a circular dichroism (CD) analysis confirmed that the cysteine introduction and dye labelling have a negligible effect on the biological activity of MBP mutants ( Supplementary Fig. 2 ). To observe the real-time conformational dynamics of the MBP mutants, dye-labelled proteins were immobilized on a polyethylene glycol (PEG)-coated quartz surface through a streptavidin–biotin interaction, and were subjected to imaging using a total internal reflection fluorescence microscope ( Fig. 2a ; Supplementary Fig. 3 ). 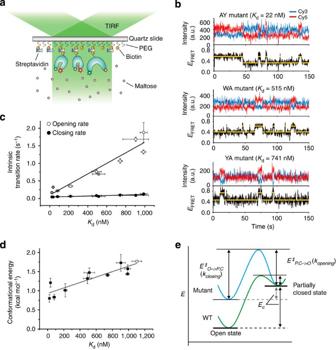Figure 2: Kinetic analysis of the intrinsic dynamics of MBP mutants through smFRET measurements. (a) Schematics of prism-type total internal reflection fluorescence (TIRF) microscopy. Immobilized proteins are excited alternatively using 532 and 633 nm lasers for Cy3 and Cy5 dye, respectively. The existence of an acceptor dye in the detected molecule is confirmed through the excitation of Cy5. (b) The representative time traces of the fluorescence intensity (top) and FRET efficiency (bottom) for MBP mutants (AY, WA and YA mutant) in the absence of a ligand. Orange lines were added as a guide to make the transition clearer. (c) The intrinsic opening and closing rates of MBP mutants were plotted with respect to the dissociation constants for maltose. Error bars represent the s.d. in duplicate experiments. (d) Conformational energies for the transition from an open to a partially closed state for the MBP mutants (▪) were calculated and plotted with the dissociation constants. The wild-type MBP (□;) was calculated based on data indicating that an intrinsic closed state is 5%. Error bars represent the s.d. in duplicate experiments. (e) An energy diagram shows two states of MBPs having intrinsic dynamics. The energy barrier between an open state and a partially closed state (EO→PC,EPC→O) determines the rate of inter-conversion (kclosing, closing rate;kopening, opening rate). MBP mutants with a higher energy level than the wild type have a lower conformational energy (Ec), and thus have less energy expenditure during the ligand-binding process. Figure 2b shows the representative time traces of the fluorescence intensity and FRET efficiency ( E FRET ) for some of the mutants in the absence of a ligand. The transitions between the two distinct conformational states were clearly detected. As previously reported [12] , the low- and high-FRET states were interpreted as open and partially closed forms, respectively. The intrinsic dynamics of the other MBP mutants could also be observed with a 100-ms time resolution in smFRET measurements ( Supplementary Fig. 4 ). Figure 2: Kinetic analysis of the intrinsic dynamics of MBP mutants through smFRET measurements. ( a ) Schematics of prism-type total internal reflection fluorescence (TIRF) microscopy. Immobilized proteins are excited alternatively using 532 and 633 nm lasers for Cy3 and Cy5 dye, respectively. The existence of an acceptor dye in the detected molecule is confirmed through the excitation of Cy5. ( b ) The representative time traces of the fluorescence intensity (top) and FRET efficiency (bottom) for MBP mutants (AY, WA and YA mutant) in the absence of a ligand. Orange lines were added as a guide to make the transition clearer. ( c ) The intrinsic opening and closing rates of MBP mutants were plotted with respect to the dissociation constants for maltose. Error bars represent the s.d. in duplicate experiments. ( d ) Conformational energies for the transition from an open to a partially closed state for the MBP mutants (▪) were calculated and plotted with the dissociation constants. The wild-type MBP (□;) was calculated based on data indicating that an intrinsic closed state is 5%. Error bars represent the s.d. in duplicate experiments. ( e ) An energy diagram shows two states of MBPs having intrinsic dynamics. The energy barrier between an open state and a partially closed state ( E O → PC , E PC → O ) determines the rate of inter-conversion ( k closing , closing rate; k opening , opening rate). MBP mutants with a higher energy level than the wild type have a lower conformational energy ( E c ), and thus have less energy expenditure during the ligand-binding process. Full size image We determined the intrinsic opening and closing rates of the mutants using a dwell time analysis ( Supplementary Table 1 ; Supplementary Figs 5–7 ). As shown in Fig. 2c , the intrinsic opening rates of the mutants significantly varied, showing a linear relation with the dissociation constants ( K d ); a mutant with a higher dissociation constant exhibited a higher intrinsic opening rate. On the other hand, the intrinsic closing rates of the mutants showed a much smaller variation than the intrinsic opening rates. To examine the relationship between the conformational energy and the binding affinity, we determined the conformational energy required for a structural transition from an open to a partially closed state for each mutant, as described in our previous work [12] . The conformational energies of the MBP mutants had a correlation with the dissociation constants; a mutant with a lower dissociation constant showed a lower conformational energy ( Fig. 2d ). This result supports the view that the intrinsic dynamics reduces the energy expenditure required for a conformational transition that occurs on ligand binding. The crystal structures of MBP in both open and closed forms revealed that Ile329 and Ala96 are tightly packed in an open state, but are exposed to a solvent in a closed state. Therefore, mutations in the hinge region of MBP are thought to perturb the energy of the ground open states [13] , [15] , thereby altering the dynamic properties of the protein. Compared with the wild type, a mutant with an increased energy level in an open substate has a lower structural energy cost ( E c ) for transition to a partially closed state, but has a higher energy barrier ( E ‡ PC→O ) for transition to an open state from a partially closed state, leading to a slower opening rate ( Fig. 2e ). Our kinetic analysis indicates that the transition state of the conformational dynamics is destabilized by the same amount. Conformational dynamics of ligand-bound MBPs To examine the effect of a ligand on the intrinsic conformational dynamics, we performed smFRET experiments at varying maltose concentrations. The closed state became more populated at increasing maltose concentrations ( Fig. 3a ). The slope of the linear correlation represents how sensitively the intrinsic conformational dynamics is affected by a ligand. A kinetic analysis revealed that the closing rates linearly increase with the ligand concentration, whereas the opening rates remain more or less the same over a wide range of maltose concentrations ( Fig. 3b ). No mutant exhibited a ligand dependency of the opening rate ( Fig. 3b ; Supplementary Figs 6–8 ), which indicates that the ligand dissociation is solely determined by the intrinsic conformational dynamics of the MBPs. Interestingly, however, the slope of the closing rate varied between mutants; MBP mutants with smaller dissociation constants had steeper slopes ( Fig. 3c ). On the basis of single-molecule maltose titration experiments ( Supplementary Fig. 8 ), the dissociation constants of maltose for different MBP mutants were determined ( Supplementary Table 2 ). The results show that they are similar to those determined through ITC measurements. The maltose-binding energies were determined from the dissociation constants of MBP mutants ( Table 1 ) and their conformational energies ( Fig. 2d ). Quite unexpectedly, the hinge mutations were shown to favourably affect the ligand-binding energy ( Fig. 3d ). Using the dissociation constants based on single-molecule measurements, similar results were obtained ( Supplementary Fig. 9 ). This observation is consistent with the fact that the slope of the closing rate variation was steeper for a mutant with a low dissociation constant ( Fig. 3c ). On the basis of the results, we present an energy diagram representing the ligand binding and dissociation events of the MBPs ( Fig. 3e ). The diagram is composed of three substates, that is, ligand-unbound open, ligand-bound open and ligand-bound closed. The binding and dissociation events in the partially closed state were minor, and were therefore not considered in this study. The binding process starts in an open state. The binding of a ligand to an MBP in an open form reduces the barrier height of the conformational transition state, resulting in an acceleration of the closing rate. The fact that the opening rate of a ligand-bound closed state is similar to the opening rate of a ligand-free partially closed form indicates that the change of the MBP–ligand interaction energy during the conformational transition from an open form to a closed form is negligible compared with the conformation energy. 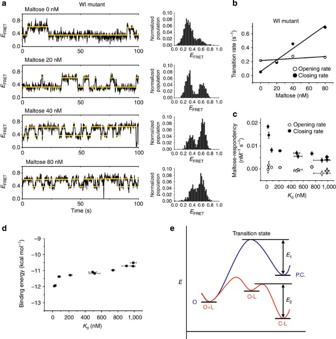Figure 3: Analysis of the MBP dynamics in the presence of varying maltose concentrations. (a) The representative time traces and FRET histogram of the WI mutant with increasing maltose concentration. Orange lines were added as a guide to make the transition clearer. (b) The closing rates of the MBP variants were plotted as a function of maltose concentration. (c) The slopes obtained from the linear fitting of the closing and opening rate inFig. 3b;Supplementary Fig. 8for MBP variants were plotted as a function of the dissociation constants. Error bars represent the s.e. in the linear fitting and s.d. in duplicate experiments for the dissociation constant. (d) The binding energies between maltose and MBP variants were plotted as a function of the dissociation constant. Error bars indicate s.d. in duplicate experiments for the dissociation constant. (e) The energy diagram shows three substates, that is, ligand-unbound open (O), ligand-bound open (O-L) and ligand-bound closed (C-L), of an MBP during binding and dissociation events. The energy barriers for a transition from a partially closed state to an open state (E1), and transition from a ligand-bound closed state to a ligand-bound open state (E2), are the same. Figure 3: Analysis of the MBP dynamics in the presence of varying maltose concentrations. ( a ) The representative time traces and FRET histogram of the WI mutant with increasing maltose concentration. Orange lines were added as a guide to make the transition clearer. ( b ) The closing rates of the MBP variants were plotted as a function of maltose concentration. ( c ) The slopes obtained from the linear fitting of the closing and opening rate in Fig. 3b ; Supplementary Fig. 8 for MBP variants were plotted as a function of the dissociation constants. Error bars represent the s.e. in the linear fitting and s.d. in duplicate experiments for the dissociation constant. ( d ) The binding energies between maltose and MBP variants were plotted as a function of the dissociation constant. Error bars indicate s.d. in duplicate experiments for the dissociation constant. ( e ) The energy diagram shows three substates, that is, ligand-unbound open (O), ligand-bound open (O-L) and ligand-bound closed (C-L), of an MBP during binding and dissociation events. The energy barriers for a transition from a partially closed state to an open state ( E 1 ), and transition from a ligand-bound closed state to a ligand-bound open state ( E 2 ), are the same. Full size image The role of conformational dynamics in a receptor–ligand interaction has been the subject of intensive studies [3] , [9] , [10] , [12] , [16] , [17] , [18] . The receptor–ligand interaction process comprises two fundamental steps, namely, the binding and dissociation of a ligand. Our recent single-molecule studies revealed that conformational dynamics plays a negligible role in the ligand-binding step of an MBP [12] . A series of MBP mutants constructed through hinge mutations were shown to have a wide range of intrinsic opening rates and dissociation constants for maltose, enabling us to investigate how protein dynamics determine the ligand dissociation, and thus the binding affinity. The hinge mutations of an MBP altered the distribution of the conformational ensemble with the ligand-binding interfaces being essentially identical. We found that the ligand–protein interaction has a negligible role in determining the opening rate of an MBP; the change in the interaction energy of MBP–maltose binding is small compared with the conformational energy. It is therefore obvious that an MBP stabilizes a weak binding complex through a structural transition to a closed form, which encloses the ligand, thereby inhibiting the ligand dissociation. Taken together, our results provided direct evidence that the intrinsic opening rate of the protein dictates the ligand dissociation, and consequently the binding affinity for a ligand. The residence time of a ligand has a significant effect on the signal transduction, regulatory processes and drug responses [2] , [3] , [4] , [5] . Ligand dissociation (or ligand residence time) is closely linked with a binding affinity for proteins. Traditionally, ligand release has been explained using a simple diffusion model [3] . With advances in experimental methods to investigate the protein dynamics, such as nuclear magnetic resonance, computational simulations and single-molecule techniques, evidence for the role of protein dynamics in ligand dissociation has been provided [9] , [10] , [19] , [20] . Recently, Carroll et al. [3] analysed the dynamics at the binding site of DHFR for a series of inhibitors with different binding affinities through nuclear magnetic resonance relaxation dispersion. Interestingly, a set of residues near the binding site were observed to undergo a millisecond-timescale switching from ground to excited conformations. The switching rate was correlated exponentially with the binding affinity of the inhibitors, which suggests that protein dynamics serve as a mechanical initiator of ligand dissociation. Our observation demonstrates that the ligand residence time can be engineered by modulating the intrinsic dynamic characteristics. From an evolutionary perspective, it is generally accepted that the biological function of a protein has been selected by evolution, and accordingly, the dynamic characteristics of a protein are the result of evolutionary selection [10] . It has been suggested that various periplasmic-binding proteins have their own dynamic characteristics along with their particular purposes [21] , [22] , [23] , [24] . MBP, for example, is involved in the uptake of various sugars in Gram-negative bacteria, and maltose uptake in vivo has been shown to be modulated by a change in the dynamic property of MBP [25] . MBP is therefore likely to have evolved to have optimal dynamics for transporting sugars for the survival of organisms. Along with other studies regarding the connection between protein dynamics and ligand dissociation or enzyme catalysis [26] , [27] , our results therefore provide direct evidence regarding the dynamics-coupled ligand dissociation at a longer timescale (sub-second to tens of seconds) with a large amplitude (domain movement and reorientation in the nm range). Allostery is ubiquitous in biology, and forms a basis for cooperativity. There has recently been growing interest in the regulation of protein functions in an allosteric manner [19] , [25] , [28] , [29] , [30] , [31] , [32] . However, the operational mechanism of the allosteric regulation remains poorly understood. For instance, in contrast to the original view that the binding of an allosteric ligand to a protein induces a structural change, it has been proposed that allosteric structural or dynamic perturbations do not induce new conformational states, but change the relative distributions of the states within the ensemble [28] . Mutations in the hinge region of an MBP, opposite the ligand-binding pocket, were proposed to induce changes in the conformational energy [12] , resulting in an allosteric modulation of the binding affinity. Our single-molecule kinetic studies provide crucial insight into the allosteric regulation mechanism of the protein function in terms of conformational dynamics; the changes in the dynamic personalities of a protein by allosteric mutations can modulate the ligand-binding affinity and vice versa, even among proteins with an identical ligand-binding interface. In contrast to the original belief, our results showed that the hinge mutations can favourably affect both the binding energy itself, and the conformational energy. It is therefore possible that long-range interactions modulate the ligand–protein interaction in an allosteric manner. The existence of conformational substates is likely to offer an alternative regulatory point by which we can regulate protein functions by modulating the dynamic characteristics. For instance, it was reported that when the equilibrium is shifted towards a closed state by closed form-specific allosteric binders, an MBP mutant has a higher maltose-binding affinity than a wild-type MBP even with a deleterious mutation in the binding pocket [25] . This result indicates that the affinity of a protein in vivo can be dynamically controlled, even without mutations in the protein itself, by introducing an external effector to modulate its activity. We therefore believe that this strategy can be a supplementary method or an alternative to traditional engineering methods in modulating protein–ligand interactions for molecular engineering and functional regulation. The function of a protein depends on the binding and dissociation of a ligand, and the binding affinity (or ligand residence time) has a critical effect on the regulatory processes, enzyme turnover and drug efficacy. Recent studies have shown the prominent roles of protein dynamics in many biological processes including protein–ligand interactions. Understanding the fundamental mechanisms of ligand binding and dissociation will deepen our knowledge on the protein functions and their regulations. In this regard, the present study demonstrating the interplay between conformational dynamics and binding affinity provides crucial insight into an understanding of biological processes, and can aid in the design of drugs and proteins with greater potential. Materials Cy3-maleimide and Cy5-maleimide were purchased from GE Healthcare. The maltose and HABA/avidin reagents were purchased from Sigma. The Streptavidin was provided by Invitrogen. All other reagents were of analytical grade. Protein expression and purification A gene for an MBP was cloned from the pMAL-p2X vector. The BirA gene coding for the biotin acceptor peptide (15 residues) was attached at the N terminus of the MBP gene for biotinylation. The resulting MBP gene in plasmid pET21a (Novagen) had a hexahistidine tag at the C terminus. For the construction of MBP variants with different binding affinities for maltose, various types of amino-acid residues were introduced into Ala96 and Ile329, and both Lys34 and Arg354 were changed to cysteine for dual labelling with a FRET pair (Cy3 and Cy5) ( Supplementary Table 3 ). Newly constructed vectors containing MBP variants were transformed into Escherichia coli BL21 (DE3) cells harbouring a biotin ligase gene in the pProTrc vector. Protein expression was induced with 0.5 mM isopropyl β- D -1-thiogalactopyranoside and 50 μM D -biotin at 18 °C. Biotinylated MBP variants were purified using a Ni-NTA superflow matrix (Qiagen) followed by gel filtration chromatography using a phosphate-buffered saline (PBS) buffer (137 mM NaCl, 2.7 mM KCl, 10 mM Na 2 HPO 4 , 1.76 mM KH 2 PO 4 and pH 7.4). The protein concentration was measured using the Bradford method, and HABA/avidin reagents (Sigma) were used to quantify biotin-conjugated protein [12] , [33] . Dye labelling MBP variants containing two Cys residues were labelled with Cy3- and Cy5-maleimide dyes. The proteins were incubated with a 100-fold molar excess of Tris (2-carboxyethyl) phosphine for reducing the inter-molecular disulphide bond, and then mixed with a 20-fold molar excess of two dyes for 2 h at room temperature. Dual-labelled MBPs were separated from the un-reacted dyes using a PD-10 column with a PBS buffer. The fraction of the dual-labelled MBP was estimated by measuring the absorbance at 280, 552 and 650 nm. CD analysis Wild-type MBP and its variants were analysed using JASCO J-815 with a quartz cell with a path length of 0.1 mm. CD spectra of 1 mg ml −1 MBPs were taken between 250 and 200 nm with a 1-nm increment, and a background spectrum with a free buffer (PBS) solution was subtracted. ITC All ITC experiments were carried out using an ITC200 system (Microcal) at 7.0 °C. A solution of 20 μM maltose in PBS was titrated with 200 μM of each MBP variant for a 2-min injection duration to return the titration peak to the baseline. After fitting the integrated endothermal peaks, the K d values were determined using a software provided by the supplier. smFRET experiments SmFRET measurements were conducted based on our previous work [12] with minor modifications. Briefly, to prevent the non-specific binding of proteins on the surface, the quartz slides and coverslips were cleaned, followed by PEGylation with PEG and biotin-PEG (Laysan Bio) [34] . A sample chamber was created by combining a cover slip and quartz slide with double-sided adhesive tape. The proteins were immobilized on the surface through the successive addition of 200 μg ml −1 of streptavidin and 0.5–2.0 nM of biotinylated MBPs in a TN buffer (10 mM Tris–HCl, pH 8.0 and 50 mM NaCl). A protocatechuic acid/protocatechuate-3,4-dioxygenase oxygen-scavenging system [35] and a blinking suppressant, Trolox [34] , were used to reduce the photobleaching and blinking of the dyes. Single-molecule fluorescence images were taken of the imaging buffer (10 mM Tris–HCl, pH 8.0, 50 nM protocatechuate-3,4-dioxygenase, 2.5 mM protocatechuic acid and 1% (v/v) Trolox) in the presence or absence of maltose using a home-built prism-type total internal reflection fluorescence microscope at 23 °C. The alternative excitation of Cy3 and Cy5 was performed using a 532 and 633-nm laser with a mechanical shutter, respectively [36] . The fluorescence signals of the two dyes were collected using a water immersion objective lens (UPlanSApo × 60; Olympus), and filtered through 532 nm and 633 nm notch filters (NF03-532E-25 and NF01-633U-25; Semrock). The fluorescence signals were then separated using dichroic mirrors (635dcxr; Chroma Technology) and detected through an electron-multiplying charged-coupled-device (Ixon DV897; Andor). Analysis of smFRET data From the images of an acceptor detection channel, a few hundred single-molecule spots were picked by alternating the 532 and 633 nm laser excitations to collect only the dual-labelled proteins from the heterogeneous populations. Using custom made IDL (Exelis Visual Information Solutions) software, only dual-labelled proteins were picked from the detected images. The intensity traces of Cy3 and Cy5 were analysed using a custom made Matlab (MathWorks) script. The FRET efficiencies were calculated using the intensity-based equation using the donor ( I D ) and acceptor ( I A ) fluorescence intensities, that is, I A /( I A + I D ) [34] . To calculate the kinetic rates of the state change, the dwelling time of each state in the real-time traces was measured in the absence or presence of varying ligand concentrations. The data were fitted with a single exponential decay function, and the coefficients of the function were used for calculating the kinetic rates [12] . Determination of the dissociation constant As described in our previous work [12] , dissociation constants ( k d ) for MBP mutants were obtained from the following equation: where is the intrinsic closing rate and is the intrinsic opening rate. The accelerated closing rates ( k closing ) are given by where α is the slope of closing rate as a function of maltose concentration ( L ). Calculation of the conformational and binding energies The conformational energy ( E c ) required for the transition from an open state to a partially closed state was calculated from the probability of an intrinsic closed state, as described in our previous work [11] . In statistical mechanics, the relative probability of a state is determined based on a Boltzmann factor of the state, from which the free energy of a partially closed state relative to an open state was calculated. The relative probability was directly obtained from smFRET experiments for the MBP variants, whereas a reported value of 5% was used for a wild-type MBP [37] . The binding free energy ( ΔE , the energy difference on taking a ligand from a solution and placing it on a protein) was determined using the following equation: which was obtained as described in our previous work [12] . How to cite this article: Seo, M.-H. et al. Protein conformational dynamics dictate the binding affinity for a ligand. Nat. Commun. 5:3724 doi: 10.1038/ncomms4724 (2014).